GermlineTP53mutations undergo copy number gain years prior to tumor diagnosis 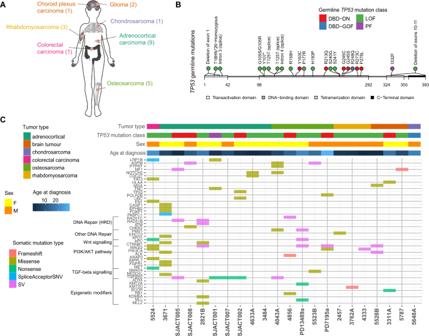Fig. 1: The mutational landscape ofTP53-germline mutant childhood tumors. ATP53-germline mutant tumors included in study. (#) indicates number of tumors of each tumor type.BLocation of germline mutations inTP53gene, colored by functional impact. DBD-DN DNA binding domain-dominant negative, DBD-GOF DNA binding domain- gain of function, LOF loss of function, PF partial function.CTop: Clinical covariates (tumor type, germlineTP53mutation class, sex, age), Bottom: Predicted somatic driver mutations arranged by pathway and colored by type of mutation. Li-Fraumeni syndrome (LFS) is a hereditary cancer predisposition syndrome associated with germline TP53 pathogenic variants. Here, we perform whole-genome sequence (WGS) analysis of tumors from 22 patients with TP53 germline pathogenic variants. We observe somatic mutations affecting Wnt, PI3K/AKT signaling, epigenetic modifiers and homologous recombination genes as well as mutational signatures associated with prior chemotherapy. We identify near-ubiquitous early loss of heterozygosity of TP53 , with gain of the mutant allele. This occurs earlier in these tumors compared to tumors with somatic TP53 mutations, suggesting the timing of this mark may distinguish germline from somatic TP53 mutations. Phylogenetic trees of tumor evolution, reconstructed from bulk and multi-region WGS, reveal that LFS tumors exhibit comparatively limited heterogeneity. Overall, our study delineates early copy number gains of mutant TP53 as a characteristic mutational process in LFS tumorigenesis, likely arising years prior to tumor diagnosis. Li-Fraumeni syndrome (LFS) is an autosomal dominant cancer predisposition syndrome characterized by the early onset of a spectrum of childhood and adulthood cancers including adrenocortical carcinomas, soft tissue sarcomas, osteosarcomas, brain tumors and pre-menopausal breast cancers [1] , [2] . More than 70–80% of patients who fit the clinical definitions of LFS harbor pathogenic germline variants (mutations) in TP53 , a tumor suppressor gene which coordinates the cellular response to DNA damage [3] , [4] , [5] , [6] . Current LFS patient management focuses on identifying and treating tumors at early stages through intensive multimodal surveillance protocols [7] . It is thought that TP53 mutation carriers may be at a greater risk of developing radiation and chemotherapy-induced second primaries. However, there is little direct evidence to confirm this and while caution is recommended in the use of radiation in LFS patients, current treatment protocols for LFS-associated tumors do not differ from that of their sporadic counterparts. Several studies have shown an elevated number of structural variants in tumors from LFS patients, as well as frequent chromothripsis, and an enrichment for single base substitution (SBS) mutational signatures SBS3, SBS8 and SBS13 [8] , [9] , [10] . Critical questions remain unanswered. What are the recurrent second hits following germline mutation of TP53 ? How do LFS tumors evolve? How do the effects of treatment manifest in subsequent primary tumors in these patients? In this study, we perform whole-genome sequence (WGS) analysis on 22 tumors, across a range of LFS-spectrum tumor-types, from pediatric and young adult germline TP53 mutation carriers. We observe frequent mutation of genes involved in Wnt signaling, PI3K/AKT signaling, epigenetic modifiers and homologous recombination (HR). Mutational signatures consistent with HR-deficiency are found in 4/4 tumors with somatic HR pathway mutations. We identify frequent chromothripsis and almost ubiquitous loss of heterozygosity (LOH) of TP53 , with a gain of the mutant allele, which we time using clock-like mutational signatures to have occurred years before tumor diagnosis, likely in utero or early infancy. We found that TP53 LOH occurs much earlier in mutational time in tumors arising in patients with a germline TP53 mutation vs tumors with a somatic TP53 mutation. We confirm our finding that TP53 LOH is an early ubiquitous process in Li-Fraumeni syndrome, using primary fibroblast cell lines generated from skin biopsies of TP53 mutation carriers. These primary fibroblast cell lines spontaneously underwent LOH within months of cell culture, gaining additional copies of mutant TP53 . High levels of mutant p53 specific expression are detected in individual cells as early as 12 passages. Using bulk and multi-region WGS (46 total tumor regions), we reconstruct phylogenetic trees of tumor evolution, observing tumors arising in patients with a germline TP53 mutation to exhibit proportionally larger sets of early truncal mutations. Overall, our study delineates early TP53 LOH copy number gains in association with a later set of cooperating clonal somatic driver mutations as being the predominant mechanism of tumor evolution in our cohort of germline TP53 mutation carriers. Many of the somatic driver mutations are of clinical relevance and we present preliminary data from an ongoing prospective sequencing study suggesting precision-oncology may have particular clinical utility in the care of LFS patients. The genomic landscape of LFS-associated tumors The primary genetic cause of Li-Fraumeni syndrome has been known for 30 years: germline mutations in TP53 have been found in >70–80% of cases [11] . The somatic mutational events which cooperate with these germline TP53 mutations, however, remain unclear. To address this, we performed somatic WGS analysis of 22 tumors (46 tumor regions) from childhood and young-adult patients [age 0–28, median age: 7.5] with confirmed pathogenic germline TP53 mutations (Fig. 1A, B ; Data S1 ). The samples analyzed spanned a range of LFS-spectrum tumor types (adrenocortical tumors [ACC], n = 9; osteosarcoma [OS], n = 5; rhabdomyosarcoma [RMS], n = 3; low grade gliomas [LGG], n = 2; choroid plexus carcinoma [CPC], n = 1; chondrosarcoma [CHS], n = 1; colorectal carcinoma [CRC], n = 1) (Fig. 1A ; Data S1 ). Patients harbored a diverse set of germline TP53 mutations. Twelve patients harbored heterozygous loss of function (LOF) mutations, 6 had heterozygous dominant negative mutations in the DNA binding domain (DBD-DN), one had a heterozygous partial function (PF) mutation and one had a heterozygous gain of function mutation in the DBD domain (DBD-GOF) (Fig. 1B ). Notably, one patient (4333) presented with a homozygous TP53 frameshift mutation (T18Hfs*26) related to consanguinity [12] , and a second (5526B) presented with two distinct TP53 variants at the same base position in addition to a wildtype allele (G105S/G105R/WT), possibly due to a simultaneous mutation event during embryogenesis or aberrant clonal expansion [13] , [14] (Fig. 1B , Fig. S1 , Data S3 , Data S4 ). Fig. 1: The mutational landscape of TP53 -germline mutant childhood tumors. A TP53 -germline mutant tumors included in study. (#) indicates number of tumors of each tumor type. B Location of germline mutations in TP53 gene, colored by functional impact. DBD-DN DNA binding domain-dominant negative, DBD-GOF DNA binding domain- gain of function, LOF loss of function, PF partial function. C Top: Clinical covariates (tumor type, germline TP53 mutation class, sex, age), Bottom: Predicted somatic driver mutations arranged by pathway and colored by type of mutation. Full size image We began our analysis on the LFS tumor cohort by investigating somatic driver mutations occurring in addition to TP53 . Analysis of predicted driver mutations including SNVs, indels and structural variants (SVs) revealed several recurrently mutated genes and pathways including ATRX ( n = 4), CTNNB1 / APC ( n = 4), homologous recombination ( CHEK2, RAD51B, RAD51C ) ( n = 4) and PI3K/AKT signaling ( PI3KCA, INPPL1 , etc.) ( n = 8). (Fig. 1C ). The ATRX mutations were predicted loss of function variants and these tumors displayed evidence of elongated telomeres, as determined by Telseq analysis comparing tumor vs matched normal blood. This represents an alternative lengthening of telomere phenotype, consistent with ATRX inactivation (Fig. S2 ) [15] . The mutational processes operating in LFS-associated cancers To explore the processes causing accumulation of somatic mutations in LFS tumors, we performed mutational signature analysis using SigProfiler [16] . We identified 18 single nucleotide base substitution (SBS) signatures in the cohort. SBS1 (clock-like signature associated with spontaneous 5-methylcytosine deamination) and SBS5 (clock-like signature of unknown etiology) were present in all tumors (Fig. 2 ) and were found to correlate with patient age as has been shown previously in many adult tumor types (Fig. S3 ) [17] . SBS2 and 13 (APOBEC activity) were present in 16/22 tumors and were especially prevalent in ACCs. SBS21 (MMR-deficiency) was present in one tumor (3671), which was one of the two tumors with a mutation burden over 5 mut/Mb. SBS3 (homologous recombination-deficiency (HRD)/BRCA) was present in 10 tumors, including 5 of the 9 ACCs and all 4 of the tumors with mutations in an HR pathway gene. A high frequency of deletions at sites of microhomology, a hallmark of HRD, was also found in these tumors (Fig. S4). SBS18 (reactive oxygen species) was present in 9 tumors, although generally in low proportions. SBS88, a signature recently identified as being caused by the genotoxin, colibactin, produced by pks + E. coli , was identified in the colorectal cancer, 5524 [18] . SBS8, 16, 17a, 17b, 30, 38, and 41 (all of unknown etiology) were also present in one or more tumors. Interestingly, the two tumors with high mutation burdens (tumors: 3671 and 5524) exhibited large contributions of SBS35 (platinum therapy). Dinucleotide base substitution (DBS) analysis revealed that both tumors had large numbers of CT > AA/AC mutations in a pattern consistent with COSMIC dinucleotide base substitution DBS5 (Fig. S5 ). This pattern has previously been associated with platinum drug treatment of human cancer as well as in cell lines treated with carboplatin and cisplatin in vitro [19] , [20] . Interestingly, although sequenced samples from tumor 5524, a CRC, and 3671, an ACC, were obtained before any treatment had been initiated for these tumors, both patients had previously been diagnosed with separate primaries (OS and CPC, respectively) and had received cisplatin and/or carboplatin therapy >5 years before diagnosis of the later primary CRC and ACC. These results indicate that platinum-based chemotherapy treatment for LFS tumors can result in a substantial number of mutations detected in subsequent primary tumors and may directly contribute to their genesis. Fig. 2: The mutational signatures of TP53 -germline mutant childhood tumors. Top: Clinical and genomic features of the tumors (number of structural variants (SVs), presence of chromothripsis, prior platinum treatment, HRD pathway mutation). Bottom: SBS mutational signatures corresponding to COSMIC mutational signatures V3.2, scaled by mutation burden in tumor (above) and scaled to proportions of 1 for each tumor (below). X-axis depicts individual tumors. Source data are provided as a Source Data file. Full size image TP53 mutant copy number gains, frequently associated with LOH, are an early and defining feature of LFS tumors The most common recurrent somatic event observed across the cohort was LOH of the TP53 locus, which occurred in 18/21 (86%) of the tumors that harbored heterozygous germline TP53 mutations. Thus, the rate of TP53 LOH in LFS tumors is substantially higher than previously reported [21] .This could be due to our focus on pediatric cancers and/or our use of the more sensitive method of WGS as compared to Sanger sequencing approaches used by others. Interestingly, the one sample with a TP53 gain of function germline mutation (R248Q), was not observed to have undergone TP53 LOH. Notably, in only one case, an ACC, was a somatic point mutation in TP53 identified, suggesting that point mutations are not a common mechanism by which these tumors lose wildtype p53 function. Also, as previously reported in LFS tumors [10] , [22] , chromothripsis was prevalent in our cohort (10/22 cases) (Fig. 2 ). Given the unexpectedly high rate of TP53 LOH across our cohort, we sought to investigate this phenomenon in greater detail. To begin with, we classified TP53 LOH according to the major and minor allele copy number as well as the size of the event (segmental, whole chromosome 17). LOH can occur with no change of copy number in the mutant allele of TP53 (LOH), a single duplication of the mutant TP53 allele (copy-neutral LOH), or multiple gains of the mutant TP53 allele (copy-gain LOH). Our classification of TP53 copy number revealed a diversity of states, ranging from whole chromosome copy-neutral LOH ( n = 8), segmental copy-neutral LOH ( n = 7), whole chromosome copy-gain LOH ( n = 1), and segmental copy-gain LOH ( n = 2) suggesting that TP53 LOH occurs via an array of mechanisms in LFS patients (Fig. 3A ). Surprisingly, none of the tumors exhibited LOH in the absence of a gain of the mutant allele of TP53 . Of the three tumors in which we did not observe LOH, 2 had an allele-specific copy number gain of the mutant allele, with retention of the wildtype allele. Overall, 21/22 (95%) tumors exhibited a copy-number gain (2–3 copies) of a mutant TP53 allele. This was supported in all cases by an increase in the variant allele fraction (VAF) of the TP53 mutation in the tumor versus germline (Fig. S6 ). Of note, although complex chromothriptic events were common in our cohort, the TP53 locus was not involved in these events, suggesting that secondary hits to TP53 develop through other mechanisms. Fig. 3: TP53 LOH is an early event in the lifetime of LFS patients. A Copy number of somatic individual mutations (black and gray points) on chromosome 17 across cohort of TP53 -germline mutant tumors. Each black box represents chromosome 17 for one tumor. X-axis for each black box is the position on chromosome 17; Y -axis shows the copy number. Red and green bars are major and minor copy number. Gray points are colored by probability of contributing to SBS1 (clock-like signature). Colored squares at top represent CN state of TP53 . CG copy gain. CN copy number. B Number of aging associated mutations (SBS1 or SBS5) occurring before (blue bar) and after (red bar) TP53 CN-LOH. X-axis depicts individual tumors. Y -axis depicts number of aging associated mutations. Source data are provided as a Source Data file. Full size image The frequent gain of TP53 -mutant copies presents an opportunity to time this event in the molecular evolution of the tumor. Clonal mutations occurring before duplication of the mutant chromosome are expected to have an average copy number of 2, whereas those occurring after the event should have an average copy number of 1 (or less if subclonal). Previous reports using this approach have indicated somatic copy number events may occur many years or even decades prior to tumor diagnosis [23] . To time TP53 LOH we focused on germline TP53 mutant tumors in which copy neutral LOH of the entire chromosome 17 had occurred (i.e. those in which we observed a loss of the wildtype TP53 -containing chromosome and single copy gain of the chromosome harboring the mutant allele). To estimate timing of LOH in these samples in the lifetime of the patient, we determined the mutation copy number of mutations on chromosome 17 (Fig. 3 ). We observed that in all cases, the majority of mutations had a copy number near 1, and were predicted to occur after duplication of the TP53 -mutant copy of chromosome 17. Since SBS1 mutations accumulate as a clock-like signature over time, we sought to quantify the number of mutations along chromosome 17 contributing to SBS1 in tumors which had undergone CN-LOH. Specifically, we determined the probability for each mutation, being due to SBS1, based on its trinucleotide sequence (Fig. 3A ). Strikingly, the vast majority of mutations due to the SBS1 for all tumors with CN-LOH of chromosome 17 occurred after duplication of the mutant containing chromosome. Thus, CN-LOH occurs many years before tumor diagnosis, likely in utero or early in life (Fig. 2B ). Having established that TP53 LOH occurs early in these tumors, we next compared the timing of TP53 LOH in our cohort to what occurs in spontaneous tumors in non-LFS individuals. We applied MutationTimeR, an algorithm that determines the fraction of mutations occurring before copy-gain events [24] , to the TP53 CN-LOH events in our LFS cohort and all TP53 CN-LOH events in the somatic TP53 mutant PCAWG dataset. An example of MutationTimeR applied to one of the LFS tumor samples is shown in Supplementary Fig. 7 . We found that the TP53 LOH occurred earlier in mutational time in LFS tumors compared to that seen in somatic TP53 mutant samples in PCAWG (Fig. 4A ). In the LFS tumors, TP53 LOH usually occurred in the first 25% of mutational time, whereas in the somatic TP53 mutant tumors TP53 LOH usually occurred in the second half of mutational time (Fig. 4A ). There was no significant effect of age of tumor diagnosis on mutational timing of TP53 LOH (Fig. 4B ). Interestingly, the timing did differ by tumor type within the LFS cohort (Fig. 4C ). The adrenocortical carcinomas had the earliest timing of TP53 LOH, with almost no mutations occurring before this event. On the other hand, the osteosarcomas had the latest timing of LOH, with almost 50% of mutations occurring before LOH. Fig. 4: TP53 LOH occurs earlier in mutational time in LFS tumors than in TP53 somatic mutant tumors. A LFS tumors (left) and PCAWG TP53 somatic mutant tumors (right) plotted by TP53 LOH mutation time ( Y -axis). Wilcoxon 2-tailed p -value shown. Boxplots show quartiles with whiskers representing 1.5x interquartile range. N = 501 biologically independent samples from distinct patients. B Age at diagnosis vs TP53 LOH mutation time for PCAWG TP53 somatic mutant tumors ( Y -axis). Pearson correlation shown. Shaded area represents 95% CI. C TP53 LOH mutation time by tumor type and LFS status. Red points are LFS tumors, blue points are somatically mutant tumors in PCAWG. Boxplots show quartiles with whiskers representing 1.5x interquartile range. Source data are provided as a Source Data file. Full size image Our findings suggest that copy number gains of mutant TP53 are an early and near-ubiquitous event in LFS patients’ tumors. Given this, we sought to determine if we could detect mutant TP53 copy number gains and/or other mutational events not only in tumors, but also in non-malignant cells from LFS patients. To investigate this, we analyzed normal colonic tissue taken during the colorectal cancer surgery for tumor 5524, performing ultra-deep whole exome sequencing (5,517x mean depth) as well as ddPCR of all driver mutations identified in the tumor, in addition to two heterozygous SNPs at the TP53 locus. We were unable to identify driver mutations from the tumor in the nonmalignant tissue and the sensitivity of ddPCR was unable to resolve a significant shift in the allelic ratio (from 50:50) in the TP53 -associated heterozygous SNPs (Fig. S8 ). This analysis was limited by our sensitivity to detect rare events in an analysis of a large number of non-clonal cells. To overcome this challenge and characterize the frequency and timing of spontaneous TP53 LOH in LFS patients we leveraged the unique biology of LFS patient derived fibroblasts, which spontaneously immortalize in culture [25] . We passaged primary fibroblast cell lines obtained from skin biopsies of patients with germline R248Q TP53 mutations. We then performed WGS at an average of 40X depth on early (12–14 passages) and late primary fibroblast passages (37–38 passages) as well as on matched blood-derived DNA. In 2 of the 3 patients’ fibroblasts analyzed, we identified copy number gains of the mutant allele of TP53 by WGS in the late passage (Fig. S9 ). In the first cell line we observed multiple copy gains of the mutant allele of TP53 in 17p as well as a single copy gain of 10q. In the second cell line we observed a large number of copy number changes across the genome with a genome duplication event resulting in 4 copies of the mutant allele of TP53 and 2 copies of the wildtype allele. The third cell line showed a quiet diploid genome, with no evidence of copy number changes of TP53 by WGS. To more precisely determine LOH timing and whether TP53 LOH was present in a subset of cells at earlier passages, but simply not detected by WGS, we performed immunofluorescence using a mutant p53 specific antibody at early, middle and late passages. Previous studies have shown that mutant p53 is stabilized and accumulates in the nucleus following TP53 LOH [26] . We found that mutant p53 was expressed at high levels in individual cells as early as passage 12, subsequently becoming the dominant population of cells by passage 36 (Fig. S10 ). Overall, these results confirm that copy number gains of mutant TP53 occur spontaneously in LFS patient cells and can readily outcompete diploid clones in a small number of generations. These results align with our model in which TP53 mutant copy number gain is an early spontaneous event in LFS tumorigenesis. The clonal evolution of LFS tumors is marked by a large clonal population of mutations We next sought to investigate the role of TP53 mutations in shaping childhood cancer evolution by examining the clonality of somatic mutations. To do this we analysed the TP53 germline-mutant cohort alongside TP53 somatic-mutant ( n = 15) and TP53 -wildtype ( n = 33) tumor samples, as part of the SickKids Cancer Sequencing (KiCS) childhood precision medicine program [27] . These tumors were selected to match the LFS tumor cohort. Using PhyloWGS in single-sample mode we reconstructed the phylogenetic trees for all tumors. The proportion of clonal versus subclonal SNVs and CNVs differed markedly based on TP53 mutation status (Fig. 5A ). When comparing the proportion of SNVs and CNVs in the major clone to those which were subclonal, TP53 germline-mutant and TP53 somatic-mutant tumor samples exhibited a significantly higher proportion of mutations which were clonal as compared to TP53 wildtype tumors (Fig. 5A, B ). Fig. 5: TP53 mutant tumors have high proportion of clonal mutations. A Boxplots showing proportion of SNVs per tumor (colored circles), which are clonal. Wilcoxon 2-tailed p -value shown. Colors indicate tumor type. Boxplots show quartiles with whiskers representing 1.5x interquartile range. N = 47 biologically independent samples from distinct patients. X -axis depicts TP53 status, Y -axis depicts proportion of SNVs which are clonal. B Boxplots showing proportion of CNVs per tumor (colored circles), which are clonal. Wilcoxon 2-tailed p -value shown. Boxplots show quartiles with whiskers representing 1.5x interquartile range. Colors indicate tumor type. -axis depicts TP53 status, Y -axis depicts proportion of CNVs which are clonal. C , D Phylogenetic reconstructions of LFS tumors using multiregion WGS ( C ) Circle plots, with subclonal cluster number on X -axis and tumor region on Y -axis. Circles are colored by tumor region. Circle diameter corresponds to cancer cell fraction (CCF) for each cluster for each tumor region. D Phylogenetic tree reconstructions of each multiregion sequenced tumor with colors corresponding to tumor region, numbers corresponding to cluster number and annotated with location of driver mutations. Source data are provided as a Source Data file. Full size image To understand how the timing of mutations in LFS tumors was reflected spatially within tumors, we performed micro-dissection of frozen tumor tissue and applied WGS to multiple regions. Using PairTree we reconstructed the tumor evolution across these multiple tumor regions in LFS (Fig. 5C, D , Fig. S11 ) and non-LFS tumors (Fig. S12 ). Interestingly, while these tumors appeared to be highly clonal when analyzing single tumor regions, we found a larger degree of subclonality when assessing SNVs and indels with multiregion sequencing. Whereas SNVs and indels displayed intratumor heterogeneity, copy number events and SVs were highly clonal even across different tumor regions. Chromothriptic events were also confined to the truncal clone, with nearly identical copy number and structural variant patterns across all tumor regions observed in these tumors (Fig. S13 ). In addition to multiregion sequencing analysis of primary tumors, we also examined the clonal evolution of tumor 3671 through analysis of 4 primary adrenocortical carcinoma tumor regions as well as a lung metastasis. Interestingly we found 4 driver mutations specific to the metastasis (Fig. 5C, D ) and copy number profile analysis showed moderate divergence of the lung metastasis from the 4 primary regions (Fig. S14 ). In this study, we present the mutational landscape of tumors arising in TP53 mutation carriers and delineate the somatic mutational processes and patterns of clonal evolution (Fig. 6A ). We observed a common set of early clonal mutational mechanisms including frequent chromothripsis, and near ubiquitous early gain of mutant TP53 . The early copy number gain associated TP53 LOH in LFS tumors relative to somatic TP53 mutant cancers may be explained by the increased selective pressures for a “second hit” to TP53 when a first hit exists from conception. Timing TP53 mutant copy gains may be a potential method for helping to determine pathogenicity of TP53 variants of unknown significance. Phylogenetic reconstruction of LFS tumors revealed an enrichment for a high proportion of clonal truncal mutations in germline TP53 mutant childhood cancers. Further studies will be needed to determine whether adult LFS cancers, especially breast cancers, bear the same genomic hallmarks of germline TP53 mutations which we find in this cohort, as well as to assess the clinical utility of precision oncology in the context of LFS. Especially important will be the evaluation of additional tumors from LFS patients who have undergone treatment for earlier tumors to assess mutational signatures associated with earlier treatments. Indeed, the identification of a cisplatin mutational signature arising from treatment of an earlier tumor, raises the possibility of in vitro studies to investigate the mutational signatures induced by various therapies on LFS-patient derived cell lines. These may be useful in delineating if and how treatment modalities should be adjusted for LFS patients to avoid additional tumors, a common question among physicians and LFS patients alike. Fig. 6: Translating our molecular understanding of LFS tumorigenesis into patient care. A Proposed model of the temporal occurrence of common events involved in the initiation and progression of tumorigenesis in patients with TP53 germline mutations. Colored arrows indicate common mutational processes operating in premalignant and malignant cells and the approximate times in tumorigenesis these processes are active. B LFS patients enrolled in the KiCS precision medicine program and their actionable findings with corresponding potential targeted therapies. Full size image Given the often poor outcomes of tumors in LFS patients using conventional treatments, we reason that these patients could be candidates for targeted therapy. In fact, in our KiCS prospective cohort study of ‘hard-to-treat’ or relapsed childhood cancer we identified 3 patients with pathogenic TP53 germline mutations (Fig. 6B ). All three patients underwent a clinically validated matched germline/somatic cancer panel analysis of >800 genes. Notably, clinically actionable results were found for all three patients, including a BRAF V600E mutation, which would make the patient a candidate for a BRAF inhibitor, hypermutation which would suggest the utility of immune checkpoint blockade and an NF1 mutation, which would make the patient a candidate for a MEK inhibitor. In our investigation, we found chemotherapy treatment of LFS tumors results in mutations detected in subsequent primary tumors. While not definitive proof of their causal role in tumorigenesis, the extent to which subsequent primary tumors are caused by previous chemotherapy (especially platinum-based) and radiotherapy in LFS patients merits further study. Our finding of a pks + E coli genotoxin signature in an LFS patient’s colorectal cancer is intriguing and suggests an opportunity for future studies to explore this as a mechanism by which LFS patients may develop such tumors. Understanding to what degree such bacteria pose an additional risk of gastrointestinal malignancies in LFS patients may be of value in designing cancer prevention strategies in this population. Our results suggest that LFS patients tumors frequently harbor targetable driver mutations, which may be ideal candidates for targeted treatments, and may be less likely to result in additional mutagenesis. Future precision oncology initiatives should investigate the use of targeted treatments early in LFS patients’ disease course. Whole genome sequencing Whole genome sequencing was performed on fresh frozen tumor-derived DNA and matched normal (blood-derived or fibroblast cell line) DNA on HiSeqX to an average depth of 40X. In addition to tumor samples sequenced in house, raw sequencing data were downloaded for 8 adrenocortical tumor-normal matched genomes [9] and 7 osteosarcoma tumor-normal matched genomes [28] and re-processed from FASTQ using in house pipelines, see below. Alignment, variant calling and filtering For driver analysis, primary mutational signature analysis and multiregion phylogenetic reconstructions FASTQ files were aligned to the hg19 reference genome using BWA-mem (v0.7.8). Duplicates were marked with Sambamba (v0.7.0), and base recalibration and realignment was performed using GATK (v4.1.3) and GATK(V3.8) respectively. Substitution and indel calls were made using MuTect2 from GATK (v4.1.9). Structural variants (deletions, duplications, inversions and translocations) were called using delly (v0.7.1 s) [29] , with a minimum of 4 discordant reads in the tumor required to call each SV. Clonal and subclonal CNVs were called using Battenberg (v3.2.2). All mutation calls (SNVs and SVs) were filtered as previously described using in house pipelines [30] . Briefly, we required a minimum depth of 10X in the tumor and normal with ≤1 reads supporting the variant in the matched normal. We also removed those variants found in a panel of normal non-neoplastic tissue sequenced ( n = 133) and analysed using the same methods, as well as those that failed at least 2 of 4 cutoffs for non-unique mapping (<70% of reads at locus map uniquely), multi-mapping clusters (seen in tumor and matched normal), excessively high mapping depth (vs the average of the normal chromosome) and those present in low complexity regions (DUST score > 60). Mutation burden was calculated per megabase, the count of all coding and non-coding variants which passed the above QC filters were divided by a genome size of 2800 Mb. For remaining analyses FASTQ files were aligned to the hg19 reference genome using BWA-mem (v0.78). Duplicates were marked with Picard (v1.1.08), and base recalibration and realignment was performed using GATK (v2.8.1). Merged in silico bulk sequencing BAMs were generated by processing together all WGS FASTQ files from multiple regions to generate a single BAM file for each tumor. BAM files generated from individual tumor regions as well as in silico merged BAMs were processed for variant calling and filtering as described below. Substitution and indel calls were made using MuTect2 from GATK (v3.4.0). Structural variants (deletions, duplications, inversions and translocations) were called using delly [29] with a minimum of 4 discordant reads in the tumor required to call each SV (v0.7.1). Clonal and subclonal CNVs were called using Battenberg v3.2.2. All mutation calls (SNVs and SVs) were filtered as previously described using in house pipelines [30] . To reiterate, we required a minimum depth of 10X in the tumor and normal with 0 reads supporting the variant in the matched normal. We also removed those variants found in a panel of normal non-neoplastic tissue sequenced ( n = 133) and analysed using the same methods, as well as those that failed at least 2 of 4 cutoffs for non-unique mapping (<70% of reads at locus map uniquely), multi-mapping clusters (seen in tumor and matched normal), excessively high mapping depth (vs the average of the normal chromosome) and those present in low complexity regions (DUST score > 60). Mutation burden was calculated per megabase, the count of all coding and non-coding variants which passed the above QC filters were divided by a genome size of 2800 Mb. Driver mutation identification SNV and indel calls passing the above filters were analysed using Cancer Genome Interpreter [31] . Variants predicted as Tier1 or Tier2 driver variants in solid tumors as well as those variants annotated as known drivers in solid tumors were classified as driver variants. Filtered structural variants, from delly, with breakpoints in known tumor suppressor genes were also included. Telomere analysis Telseq (v0.0.1), a software package designed to calculate mean telomere length from WGS data, was run on each tumor and matched normal genome [32] . TelSeq estimates mean telomere length by counting the number of reads with telomeric repeats (TTAGGG), divided by GC-adjusted coverage multiplied by the mean chromosome size. We used a read-length of 150 and a threshold of at least 12 telomeric repeats per read. This threshold has previously been found to give the best performance for TelSeq telomere length estimates generated using HiSeqX WGS data (150 bp paired-end reads) in a comparative analysis vs conventional q-PCR telomere length estimation [33] . T/N ratio was calculated by dividing the estimated telomere length (in kb) of the tumor genomes by the matched normal genome. Mutational signature analysis Mutational signature analysis was performed using SigProfiler, a non-negative matrix factorization-based tool to identify mutational signatures de novo from cancer genomic sequencing cohorts [16] . For the primary mutational signature analysis, SigProfiler was run on filtered SNV calls following HotSpot analysis to distinguish clustered and non-clustered mutations. Clustered and non-clustered mutations were analyses separately. Standard parameters for SigProfiler were used with 200 bootstrapping iterations, a minimum number of 2 signatures and a maximum number of 25 signatures. The best number of signatures selected was 7 for unclustered mutations and 3 for clustered mutations, in order to maximize minimum stability and minimize the mean L2 %. These signatures were subsequently decomposed into previously reported SBS signatures and/or novel signatures using SigProfiler [16] . For the purposes of identifying SBS1 and SBS5 mutations prior to or after whole chromosome 17 copy number gain, mutations were analyzed irrespective of clustering. 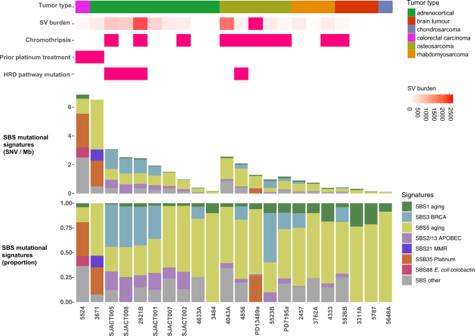Fig. 2: The mutational signatures ofTP53-germline mutant childhood tumors. Top: Clinical and genomic features of the tumors (number of structural variants (SVs), presence of chromothripsis, prior platinum treatment, HRD pathway mutation). Bottom: SBS mutational signatures corresponding to COSMIC mutational signatures V3.2, scaled by mutation burden in tumor (above) and scaled to proportions of 1 for each tumor (below). X-axis depicts individual tumors. Source data are provided as a Source Data file. The best number of signatures selected in this analysis was 8, in order to maximize minimum stability and minimize the mean L2 %. These signatures were subsequently decomposed into previously reported SBS signatures and/or novel signatures using SigProfiler, with 18 SBS signatures identified. C- > T substitutions at CpG sites, as well as all other SNVs with a >50% probability of being contributed by SBS1 or SBS5 according to SigProfiler, were used. DBS signatures were also analyzed using PhyloWGS with standard parameters. Mutation timing analysis Mutation timing was performed using SNV and battenberg copy number data (described above) with MutationTimeR version 1.0 in R.3.6.1 using default parameters (bootstrap of 10) [24] . Mutation time of the first copy number gain occurring that overlapped TP53 was used for all analyses. PCAWG data was obtained from https://dcc.icgc.org/pcawg . Subclonal analysis of individual tumor regions Filtered SNVs as described above, along with battenberg derived subclonal CNV calls were used as inputs for PhyloWGS in single sample mode [34] . A maximum of 5000 SNVs were used for each sample, with random subsampling when necessary. 10 chains were run in parallel for each sample with a burnin of 1000 iterations followed by 2500 Markov chain Monte Carlo iterations. The best tree was selected as the tree at the point of maximum density when plotting the co-clustering index versus branching degree (branching index/branching index + linearity index). The clonal fraction was determined as the number of mutations in cluster 1 divided by the total number of SNVs. Phylogenetic reconstruction of multiple tumor regions In order to explore and investigate temporal emergence of driver variants in different regions resected from single tumor samples, clonal analysis on single nucleotide variants (SNVs), small insertions and deletions (INDELs) and copy number variations (CNVs) was performed on whole-genome sequenced multi-region tumor samples using PyClone-VI, which clusters mutations based on cellular prevalence estimates using tumor purity of each sample and sex of each patient followed by inferring phylogenetic relations among these clusters using the Pairtree tool [35] . To understand and visualize mutational burden overtime, all mutations were included while calculating mutational burden for each sample and cluster. Sequencing coverage at each locus was sampled from the Poisson distribution and VAF was simulated by sampling the number of mutant reads from a binomial distribution based on the simulated coverage and success rate adjusted by purity and ploidy to give the accurate CCF distributions (clonal and subclonal). To include all samples regardless of tumor purity, no threshold for tumor purity was set during the clonal analysis. Pairtree was not only able to detect all clonal and subclonal clusters at all SNV burden levels, but it also did not assign any of the non-truncal variants to the truncal cluster, especially at this relatively low WGS coverage. This suggests that the non-truncal variants detected in the WGS dataset are not a result of noise in the data. LFS dermal fibroblast cell culture and DNA extraction Skin biopsy samples were received and dissected before being incubated with collagenase in 37 °C incubator for 1.45 h. The samples were then centrifuged at 370 g for 10 min and the supernatant was removed. Trypsin/EDTA were added to the pellets and the cells were pipetted for homogeneity and incubated at 37 °C for 30 min. These cells were then centrifuged and washed followed by incubation with alpha-MEM and 20% FCS. These cells were sub-cultured in 1 week. The cells were incubated at 37 °C in a humidified atmosphere of 5% CO2 and were maintained in DMEM (Biological Industries, Bet-Haemek, Israel) supplemented with 10% FCS and 60 mg/ml penicillin, 100 mg/ml streptomycin. The fibroblast cells were passaged for at least 37–38 passages. DNA was extracted from cell pellets by Zymo Research g-DNA mini kit as instructed by the manufacturer at early and late passages. Briefly, 50,000 cells from different passages were seeded in 6 cm plates, after the cells became confluent. The cells were then washed, trypsinized and collected in a pellet form. The pellets were then lysed using DNA lysis buffer by vortexing and incubation for 5–10 min. The cell lysates were passed through the Zymo spin column and centrifuged at 10,000 g for 1 min. The cells were washed by g-DNA wash buffer at the same speed and then eluted in 50 µl elution buffer. All steps were taken at room temperature. Finally, DNA was then sequenced and variants called as described above for tumor DNA. LFS dermal fibroblast immunofluorescence LFS fibroblasts were grown on coverslips and fixed with freshly prepared 4 % paraformaldehyde at passage 12 (early), 26 (middle) and 36 (late). Subsequently, the cells were rinsed three times with 1x PBS, washed thrice with 1x PBS with 0.5% Tween 20 and blocked overnight with 5% Bovine Serum Albumin at 4 °C. Blocking was followed by staining with the anti-mutant p53 antibody (ab32049 (Y5), abcam, 1:500 dilution) at RT in a humidified chamber for 1 h. 100ul of diluted solution, which amounts to 200 ng of primary antibody, was used per coverslip. Incubation with secondary antibody (AF488 Thermo, cat #A35552, 1:200 dilution) was also carried out under similar conditions. 100ul of diluted solution, which is equivalent to 0.5ug of secondary antibody, was used per coverslip. The cells were incubated for 5 min with 1x PBS containing 1 μg/ml DAPI, washed thrice with PBS, and mounted on microscopic slides using mounting media (Fluoromount G, Southern Biotech). 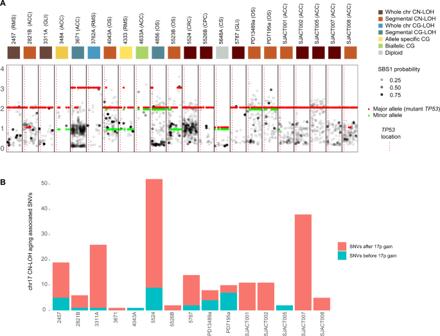Fig. 3:TP53LOH is an early event in the lifetime of LFS patients. ACopy number of somatic individual mutations (black and gray points) on chromosome 17 across cohort ofTP53-germline mutant tumors. Each black box represents chromosome 17 for one tumor. X-axis for each black box is the position on chromosome 17;Y-axis shows the copy number. Red and green bars are major and minor copy number. Gray points are colored by probability of contributing to SBS1 (clock-like signature). Colored squares at top represent CN state ofTP53. CG copy gain. CN copy number.BNumber of aging associated mutations (SBS1 or SBS5) occurring before (blue bar) and after (red bar)TP53CN-LOH. X-axis depicts individual tumors.Y-axis depicts number of aging associated mutations. Source data are provided as a Source Data file. The prepared slides were analyzed by using Zeiss LSM800 confocal laser-scanning microscope. At least 150 cells were analyzed for the experiment. Deep exome sequencing Exome sequencing was performed on DNA derived from a 6 mg sample of fresh frozen nonmalignant colonic tissue from the resection surgery for tumor 5524. 4600 ng of DNA was extracted. Exome capture was performed using Agilent SureSelect Human All Exon V5. Following exome capture, DNA was sequenced on 5 NovaSeq lanes to a depth of 5,517x for the nonmalignant colon derived DNA and a depth of 1,426x for the blood-derived DNA. 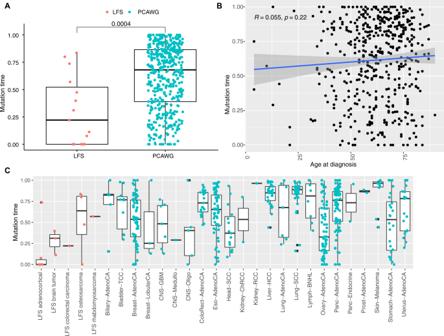Fig. 4:TP53LOH occurs earlier in mutational time in LFS tumors than inTP53somatic mutant tumors. ALFS tumors (left) and PCAWGTP53somatic mutant tumors (right) plotted byTP53LOH mutation time (Y-axis). Wilcoxon 2-tailedp-value shown. Boxplots show quartiles with whiskers representing 1.5x interquartile range.N= 501 biologically independent samples from distinct patients.BAge at diagnosis vsTP53LOH mutation time for PCAWGTP53somatic mutant tumors (Y-axis). Pearson correlation shown. Shaded area represents 95% CI.CTP53LOH mutation time by tumor type and LFS status. Red points are LFS tumors, blue points are somatically mutant tumors in PCAWG. Boxplots show quartiles with whiskers representing 1.5x interquartile range. Source data are provided as a Source Data file. Variants were called and filtered as described above for driver variant detection, with the exception of the depth filter which was required to be within 2 standard deviations of the interval depth. ddPCR analysis Digital droplet PCR analysis was performed on DNA derived from fresh frozen nonmalignant colon tissue and blood-derived DNA. ddPCR analysis was performed using the Bio-Rad QX200 systemn with custom TaqMan probes. Primers and reporter dye probes are listed in Supplementary Data 4 for each variant assessed. Consent statement Written informed consent was provided by all participants or their legal guardians, where appropriate, for this study as well as the publication of anonymized individual data. 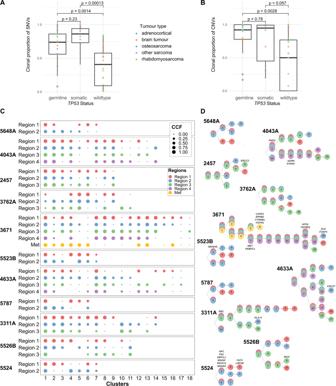Fig. 5:TP53mutant tumors have high proportion of clonal mutations. ABoxplots showing proportion of SNVs per tumor (colored circles), which are clonal. Wilcoxon 2-tailedp-value shown. Colors indicate tumor type. Boxplots show quartiles with whiskers representing 1.5x interquartile range.N= 47 biologically independent samples from distinct patients.X-axis depictsTP53status,Y-axis depicts proportion of SNVs which are clonal.BBoxplots showing proportion of CNVs per tumor (colored circles), which are clonal. Wilcoxon 2-tailedp-value shown. Boxplots show quartiles with whiskers representing 1.5x interquartile range. Colors indicate tumor type. -axis depictsTP53status,Y-axis depicts proportion of CNVs which are clonal.C,DPhylogenetic reconstructions of LFS tumors using multiregion WGS (C) Circle plots, with subclonal cluster number onX-axis and tumor region onY-axis. Circles are colored by tumor region. Circle diameter corresponds to cancer cell fraction (CCF) for each cluster for each tumor region.DPhylogenetic tree reconstructions of each multiregion sequenced tumor with colors corresponding to tumor region, numbers corresponding to cluster number and annotated with location of driver mutations. Source data are provided as a Source Data file. 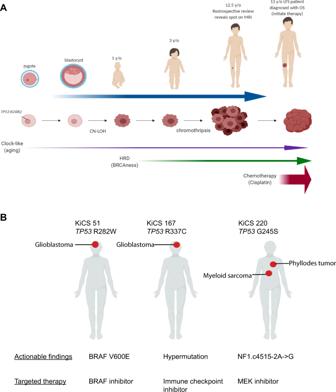Fig. 6: Translating our molecular understanding of LFS tumorigenesis into patient care. AProposed model of the temporal occurrence of common events involved in the initiation and progression of tumorigenesis in patients withTP53germline mutations. Colored arrows indicate common mutational processes operating in premalignant and malignant cells and the approximate times in tumorigenesis these processes are active.BLFS patients enrolled in the KiCS precision medicine program and their actionable findings with corresponding potential targeted therapies. No compensation was provided to participants. Informed consent to publish individual data that does not include personal health identifiers (including name, date of birth) was freely obtained. All clinical data is anonymized in the manuscript. Ethics statement The study protocol was approved by The Hospital for Sick Children Research Ethics Board and complies with all relevant ethical regulations. Reporting summary Further information on research design is available in the Nature Portfolio Reporting Summary linked to this article.